The N-terminal domains of spider silk proteins assemble ultrafast and protected from charge screening Web spiders assemble spidroin monomers into silk fibres of unrivalled tensile strength at remarkably high spinning speeds of up to 1 m s −1 . The spidroin N-terminal domain contains a charge-driven, pH-sensitive relay that controls self-association by an elusive mechanism. The underlying kinetics have not yet been reported. Here we engineer a fluorescence switch into the isolated N-terminal domain from spidroin 1 of the major ampullate gland of the nursery web spider E. australis that monitors dimerization. We observe ultrafast association that is surprisingly insensitive to salt, contrasting the classical screening effects in accelerated, charged protein interfaces. To gain deeper mechanistic insight, we mutate each of the protonatable residue side chains and probe their contributions. Two vicinal aspartic acids are critically involved in an unusual process of accelerated protein association that is protected from screening by electrolytes, potentially facilitating the rapid synthesis of silk fibres by web spiders. Orb-web-weaving spiders use seven specialized glands to spin silk threads tailored for various tasks including prey capture, reproduction and shelter [1] . Dragline silk from the major ampullate gland forms the main structural web fibre and spider’s lifeline. This thread is exceptionally tough and supersedes mechanical properties of man-made material [2] , [3] , [4] . As such, dragline silk is a focus of biotechnology and biomimetic material sciences. To mimic or reproduce spider silk, it is crucial to understand the structure–function relationship of the constituent proteins, the way they are processed in the spider’s spinneret and the interactions they form in fibres. Spider silk fibres are polymers made of protein monomers, so-called spidroins. The bulk of a spidroin sequence consists of repetitive peptide motifs of simple amino-acid composition. This central segment is flanked by non-repetitive, globular carboxy- and amino-terminal domains [3] , [5] . Spidroins have a molecular weight of about 300 kDa [1] and the non-repetitive terminal domains cover only ~10% of the sequence area but have critical roles during silk synthesis [5] . At the beginning of the spinning process, a highly concentrated solution of spidroins is stored in the ampulla of the spinning gland. During silk extrusion, spidroins pass through a tapering duct where they undergo controlled phase and structural transitions before they leave the exit spigot as solid fibre [1] . On their journey through the duct, proteins experience a series of mechanical and chemical stimuli. Shear forces align spidroins mechanically and changes of solution composition induce structural transitions [1] , [4] . The molecular basis of these transitions is only partly understood. The central sequence segment is largely disordered in the gland but forms regular and non-regular secondary structure in solid silk fibres [1] , [3] . NMR structural studies show that the carboxy-terminal domain forms a covalent, parallel homodimer that is stabilized by cross-domain disulphides, thus connecting two spidroins covalently [6] . The covalent linkage leads to dimeric strings of spidroins in solution that are terminated by the amino-terminal domains (NTDs) on opposite ends. The NTDs contain a pH-sensitive relay [7] that triggers anti-parallel homodimerization on solution acidification at physiological pH. A change of pH from 7 to 6 is induced by proton pumps located at the epithelial cells in the distal part of the spinning duct, just before spidroins leave the exit spigot as silk fibre [1] , [8] . pH-triggered NTD dimerization leads to polymerization of spidroins during their passage through the acidified assembly zone, forming supermolecules in solid silk threads [7] , [9] , [10] ( Fig. 1 ). The molecular details of this process are not yet established. 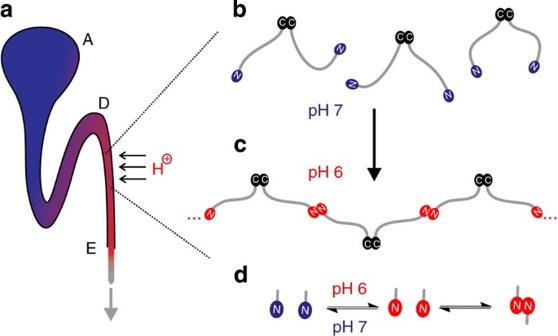Figure 1: NTD-assisted association of spidroins in web spiders. (a) Spidroins are stored in the ampulla (A) of the spinning gland. On demand, they pass through a tapering duct (D). Besides various mechanical and chemical stimuli, they experience a change of solution pH from 7 to 6 (red) in the distal part of the duct and finally leave the exit spigot (E) as solid silk fibre (grey arrow). (b) Spidroins consist of a large central, repetitive sequence motif (grey) that is flanked by small C- and N-terminal domains (displayed dimensions of the C and N domains are not to scale with the repetitive domain). The C domains form permanent, parallel dimers. (c) The N domains associate in anti-parallel orientation triggered by solution acidification, which leads to spidroin polymerization. (d) The two-step process of the pH-triggered monomer/dimer equilibrium of the N domains is illustrated. Figure 1: NTD-assisted association of spidroins in web spiders. ( a ) Spidroins are stored in the ampulla (A) of the spinning gland. On demand, they pass through a tapering duct (D). Besides various mechanical and chemical stimuli, they experience a change of solution pH from 7 to 6 (red) in the distal part of the duct and finally leave the exit spigot (E) as solid silk fibre (grey arrow). ( b ) Spidroins consist of a large central, repetitive sequence motif (grey) that is flanked by small C- and N-terminal domains (displayed dimensions of the C and N domains are not to scale with the repetitive domain). The C domains form permanent, parallel dimers. ( c ) The N domains associate in anti-parallel orientation triggered by solution acidification, which leads to spidroin polymerization. ( d ) The two-step process of the pH-triggered monomer/dimer equilibrium of the N domains is illustrated. Full size image Here we study the kinetics of association of the isolated NTD from spidroin 1 of the major ampullate gland of the nursery web spider Euprosthenops australis by means of fluorescence experiments. We engineer an extrinsic fluorescence switch that signals assembly into the NTD and emulate a change of solution pH, similar to as it happens in the spinning duct, through rapid-mixing experiments. We measure association and dissociation rate constants and their dependence on solution ionic strength (IS). We further mutate all protonatable residue side chains of the NTD to probe their contributions to assembly. Two vicinal aspartic acids emerge as critical in a pH-triggered process of accelerated protein association that is surprisingly insensitive to IS. We discuss potential implications of our findings in the rapid synthesis of silk fibres by web spiders. Design of a fluorescence reporter for NTD assembly The NTD of spidroin 1 from the major ampullate gland of the nursery web spider E. australis is a 14-kDa five-helix bundle that forms a homodimer [7] . The anti-parallel symmetry of the association interface brings the side chain of glutamine at position 50 (Q50), which flanks the interface, within 1-nm distance to itself on the opposing subunit ( Fig. 2a ). Organic fluorophores at such short distance form non-covalent dimers with substantially altered absorption and fluorescence emission characteristics [11] . We mutated Q50 to cysteine (Q50C) and chemically modified the mutant at the cysteine side chain with the thiol-reactive, red-absorbing oxazine fluorophore AttoOxa11 (F). 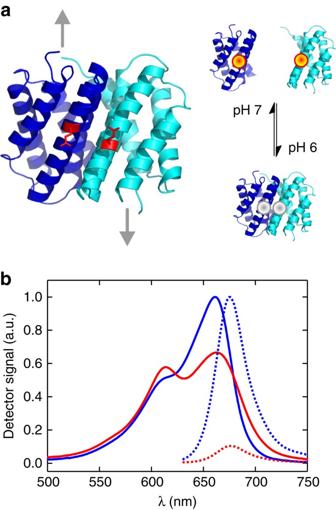Figure 2: pH-induced assembly of the NTD monitored by an extrinsic label. (a) Crystal structure of the anti-parallel NTD dimer in cartoon representation with the two subunits coloured blue and cyan (pdb id 3LR2). The positions where central spidroin sequence segments append are indicated by grey arrows. The glutamine side chains of residues Q50 (red) flank the interface and are in close proximity. Chemical modification of the cysteine mutant Q50C with the fluorophore AttoOxa11 (red sphere; NTDF) yields a probe that monitors pH-induced association through formation of H-type fluorophore dimers. (b) Steady-state absorption (solid lines) and fluorescence emission (broken lines) spectra of NTDFmeasured under monomer (pH 7.0, blue) and dimer (pH 6.0, red) solution conditions. Figure 2b shows absorption and fluorescence emission spectra of AttoOxa11-modified NTD (NTD F ) recorded in buffered solutions where the NTD is monomeric and dimeric, that is, in 50 mM phosphate pH 7.0 and in 20 mM 2-( N -morpholino)ethanesulphonic acid (MES) pH 6.0, respectively. At pH 7.0, NTD F shows the common absorption/emission characteristics of AttoOxa11. At pH 6.0, however, the absorptivity at the maximum wavelength of ~660 nm is substantially reduced with respect to the lower-wavelength absorption band at ~610 nm. These spectral changes are accompanied by a dramatic loss of fluorescence emission ( Fig. 2b ) characteristic of dimeric fluorophores in π-stacking H-type interaction geometry [11] , [12] . The dramatically changed spectral properties of H-type fluorophore dimers is explained by a delocalized electronic excitation, that is, a molecular exciton [11] . We conclude that AttoOxa11 at position Q50C yields a sensitive and specific probe for NTD dimerization. Figure 2: pH-induced assembly of the NTD monitored by an extrinsic label. ( a ) Crystal structure of the anti-parallel NTD dimer in cartoon representation with the two subunits coloured blue and cyan (pdb id 3LR2). The positions where central spidroin sequence segments append are indicated by grey arrows. The glutamine side chains of residues Q50 (red) flank the interface and are in close proximity. Chemical modification of the cysteine mutant Q50C with the fluorophore AttoOxa11 (red sphere; NTD F ) yields a probe that monitors pH-induced association through formation of H-type fluorophore dimers. ( b ) Steady-state absorption (solid lines) and fluorescence emission (broken lines) spectra of NTD F measured under monomer (pH 7.0, blue) and dimer (pH 6.0, red) solution conditions. Full size image Kinetics of NTD association and dissociation Dimerization of wild-type NTD can be followed by intrinsic fluorescence. A single tryptophan (Trp) side chain at the N terminus of the NTD is buried in the monomer but changes conformation to take a more solvent-exposed position in the dimer [13] . As a consequence, intrinsic Trp fluorescence emission is quenched on NTD dimerization [7] , [10] , [13] . We applied stopped-flow fluorescence spectroscopy to measure kinetics of NTD assembly using both intrinsic and extrinsic probes. We measured association kinetics of wild-type NTD by monitoring Trp and of NTD F by monitoring AttoOxa11 fluorescence. Samples were prepared in 10 mM MES pH 7.0 with the IS adjusted to 150 mM and rapidly mixed into 50 mM MES pH 6.0 passing through an optical stopped-flow cell. The experiment emulated conditions in the spinneret of web spiders where proton pumps in the distal part of the spinning duct initiate a change of solution pH from 7 to 6 (refs 1 , 8 ) ( Fig. 1 ). We observe kinetic transients of fluorescence quenching resulting from NTD association, which fitted well to exponential decay functions ( Fig. 3a ). 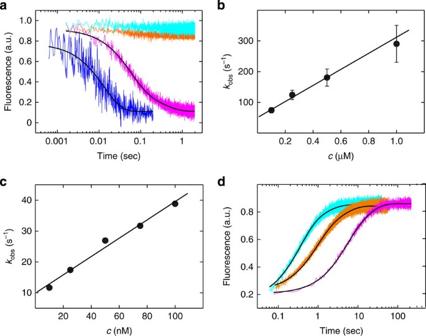Figure 3: Association and dissociation kinetics of the NTD. (a) Fluorescence transients of NTD association induced by a rapid change of solution pH from 7.0 to 6.0, measured using stopped-flow spectroscopy. Representative transients of 100 nM NTD monitored by Trp fluorescence (blue, average over seven shots) and 25 nM NTDFmonitored by AttoOxa11 fluorescence (magenta, single shot) are shown. Black lines are data fits to exponential decay functions. In addition, fluorescence transients of NTDFmutants D39N and D40N are shown in orange and cyan, respectively. (b) Observed association rate constants (kobs) obtained from Trp fluorescence of NTD and plotted versus sample concentration. The solid line is a linear data fit. Error bars are s.d. of three measurements. (c) Observed association rate constants measured from AttoOxa11 fluorescence of NTDFand plotted versus sample concentration. The solid line is a linear data fit. s.d. of three measurements were on the order of symbol size. (d) Kinetic transients of dissociation of NTDFdimers in 50 mM MES pH 6.0 measured from AttoOxa11 fluorescence using chasing experiments. Representative kinetic transients of NTDF(magenta) and mutants E84Q (orange) and R60A (cyan) are shown. Black lines are fits to exponential rise functions. Figure 3b,c shows the observed rate constants plotted versus sample concentration. All kinetic transients of association of NTD and NTD F together with data fits are provided as Supplementary Figs S1 and S2 . Observed rate constants increased linearly with sample concentration, as expected for a bimolecular event ( Fig. 3b,c ). The slopes of linear fits to the data yield association rate constants, k a , of 2.6±0.5 × 10 8 M −1 s −1 for NTD and of 3.0±0.2 × 10 8 M −1 s −1 for NTD F . The good agreement of rate constants measured from intrinsic Trp and extrinsic AttoOxa11 fluorescence shows that extrinsic modification does not perturb NTD association. Figure 3: Association and dissociation kinetics of the NTD. ( a ) Fluorescence transients of NTD association induced by a rapid change of solution pH from 7.0 to 6.0, measured using stopped-flow spectroscopy. Representative transients of 100 nM NTD monitored by Trp fluorescence (blue, average over seven shots) and 25 nM NTD F monitored by AttoOxa11 fluorescence (magenta, single shot) are shown. Black lines are data fits to exponential decay functions. In addition, fluorescence transients of NTD F mutants D39N and D40N are shown in orange and cyan, respectively. ( b ) Observed association rate constants ( k obs ) obtained from Trp fluorescence of NTD and plotted versus sample concentration. The solid line is a linear data fit. Error bars are s.d. of three measurements. ( c ) Observed association rate constants measured from AttoOxa11 fluorescence of NTD F and plotted versus sample concentration. The solid line is a linear data fit. s.d. of three measurements were on the order of symbol size. ( d ) Kinetic transients of dissociation of NTD F dimers in 50 mM MES pH 6.0 measured from AttoOxa11 fluorescence using chasing experiments. Representative kinetic transients of NTD F (magenta) and mutants E84Q (orange) and R60A (cyan) are shown. Black lines are fits to exponential rise functions. Full size image The NTD dissociation rate constant, k d , cannot be obtained under the physiologically relevant conditions at pH 6 from intrinsic Trp fluorescence. However, the engineered extrinsic probe provides a unique tool to measure k d at pH 6 using chasing experiments. We prepared dimeric NTD F in pH 6.0-buffered solution and chased one subunit off the dimer by rapidly mixing-in excess of non-modified NTD using the stopped-flow technique. Since the monomer/dimer equilibrium is dynamic and since under these conditions k a is much larger than k d , every dissociation event of dimeric NTD F results in rapid reassociation with non-modified NTD, present at excess concentration, until the equilibrium is reached and all fluorescence-quenched NTD F /NTD F dimers exchanged to fluorescent NTD F /NTD assemblies. The resulting fluorescence increase signals NTD F dissociation. Measured kinetic transients of dissociation fit well to exponential rise functions ( Fig. 3d ). To further test whether the observed kinetics truly reflected dissociation, we measured transients at various sample concentrations. The k d determined for 25, 50 and 100 nM NTD F in 50 mM MES pH 6.0 was 0.3±0.1, 0.33±0.05 and 0.26±0.05 s −1 , respectively, values which are within error. Thus, as expected, obtained values of k d are insensitive to sample concentration. The influence of IS on kinetics The monomer/dimer equilibrium of the NTD at pH 6 is dependent on IS [9] . Steady-state fluorescence emission intensities show that at low IS NTD F is dimeric but at IS>200 mM NTD F is essentially monomeric ( Supplementary Fig. S3 ). We measured k a and k d of NTD F in pH 6.0-buffered solutions of increasing IS. The results are shown in Fig. 4 . Kinetic transients together with fits to the data are provided as Supplementary Figs S4 and S5 . k a is virtually insensitive to salt. By contrast, k d increases substantially with increasing IS. In fluorescence transients of NTD F dissociation at low IS, that is, at IS<100 mM, a second kinetic phase emerges that fits to an exponential rise time, which is two- to fourfold slower than that of the main kinetic phase ( Supplementary Fig. S5 ). This additional phase may originate from the presence of low levels of NTD oligomers. Clustering fluorophores in oligomeric NTD F can undergo resonance energy transfer (homo-Förster resonance energy transfer ) leading to quenching of fluorescence and may explain the occurrence of an additional kinetic phase at low IS. In support of this interpretation, higher-order NTD oligomers have previously been observed in light-scattering experiments carried out at pH 6 (ref. 7 ). However, their presence is controversial as they have not been detected in other experimental studies [10] , [13] . 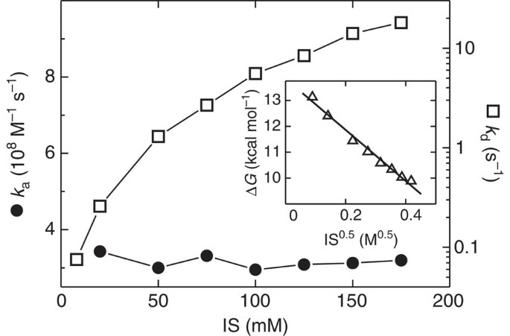Figure 4: Influence of IS on kinetics. Association rate constantska(closed circles) and dissociation rate constantskd(open squares) of NTDFmeasured at pH 6.0 and increasing IS. The inset shows the free energy of NTD dissociation calculated fromkaandkdand plotted versus the square root of IS. The solid line is a linear fit to the data. Figure 4: Influence of IS on kinetics. Association rate constants k a (closed circles) and dissociation rate constants k d (open squares) of NTD F measured at pH 6.0 and increasing IS. The inset shows the free energy of NTD dissociation calculated from k a and k d and plotted versus the square root of IS. The solid line is a linear fit to the data. Full size image From the rate constants k a and k d we calculated the equilibrium dissociation constant, K d , which is found to be in the nanomolar range and strongly dependent on IS. K d provides access to the free energy of NTD F dimerization, Δ G . All thermodynamic parameters are summarized in Supplementary Table S1 . To test whether the observed changes of k d and Δ G resulted from charge screening, we applied the Debye–Hückel formalism in the analysis of the data, which describes the activity of ions in solution [14] . Following this law, a change of Δ G originating from charge screening is proportional to the square root of IS (IS 0.5 ) [15] , [16] . We plotted Δ G of NTD assembly versus IS 0.5 and found that it changed linearly, in accord with the Debye–Hückel law ( Fig. 4 , inset). From the linear fit to the data, we extrapolate the dissociation rate constant at zero IS, k d 0 , to 0.025±0.006 s −1 . The extrapolated free energy at zero IS, Δ G 0 , is 13.8±0.2 kcal mol −1 . The influence of NTD side chain charges on kinetics The 137-residue sequence of the NTD contains a total of 12 ionizable amino-acid side chains: eight negatively charged aspartic or glutamic acids (D or E), three positively charged arginine or lysine residues (R or K) and one histidine (H). To probe their contribution to assembly, we deleted the side chain charges individually on the background of NTD F using site-directed mutagenesis. Aspartic and glutamic acids were mutated to the isosteric, non-charged asparagines and glutamines. Histidine, lysine and arginine were mutated to alanine. Kinetic transients of association and dissociation of NTD F mutants were measured in 50 mM MES pH 6.0 using stopped-flow fluorescence spectroscopy. Representative transients are shown in Fig. 3a,d . Values of k a and k d were derived in the same way as described above for the non-mutated pseudo wild-type protein. Kinetic transients of all mutants had significant amplitudes, except of D39N and D40N. D39N and D40N had virtually no fluorescence signal change and, thus, no rate constants of association or dissociation could be obtained. The values of k a and k d determined for all other mutants are shown in Fig. 5 . All rate constants together with derived thermodynamic data are provided in Supplementary Table S1 . k a was between 1–5 × 10 8 M −1 s −1 and fluctuates around the value determined for the pseudo wild-type NTD F ( Fig. 5a ). Values of k d vary with position and are significantly elevated (up to 13-fold) for all mutants ( Fig. 5b ). Mutant E119Q is an exception as it shows a fivefold decrease of k d as compared with the pseudo wild-type protein. 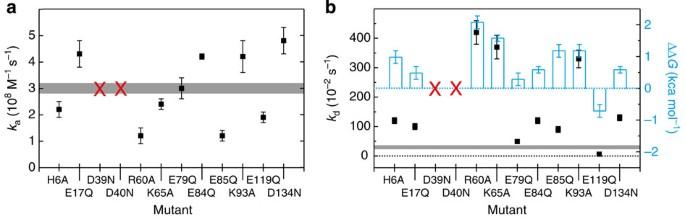Figure 5: Influence of side chain charges on kinetics. (a) Rate constants of association of NTDFand mutants thereof determined in 50 mM MES pH 6.0. Error bars are s.e. The grey horizontal line indicates the value of the pseudo wild-type protein NTDF(the width of the line represents the s.e.). (b) Rate constants of dissociation of NTDFand mutants thereof determined in 50 mM MES pH 6.0. Error bars are s.d. of three measurements. The grey and solid horizontal line indicates the value of the pseudo wild-type protein NTDF(the width of the line represents the s.d.). Open cyan bars show the changes of the free energies of dimerization for each mutant calculated fromkaandkd. Quantities for mutants D39N and D40N could not be determined because no fluorescence amplitude was detected (red X). Broken horizontal lines indicate the value zero. Figure 5: Influence of side chain charges on kinetics. ( a ) Rate constants of association of NTD F and mutants thereof determined in 50 mM MES pH 6.0. Error bars are s.e. The grey horizontal line indicates the value of the pseudo wild-type protein NTD F (the width of the line represents the s.e.). ( b ) Rate constants of dissociation of NTD F and mutants thereof determined in 50 mM MES pH 6.0. Error bars are s.d. of three measurements. The grey and solid horizontal line indicates the value of the pseudo wild-type protein NTD F (the width of the line represents the s.d.). Open cyan bars show the changes of the free energies of dimerization for each mutant calculated from k a and k d . Quantities for mutants D39N and D40N could not be determined because no fluorescence amplitude was detected (red X). Broken horizontal lines indicate the value zero. Full size image The NTD of spidroins evolved to maintain solubility of silk fibre-building blocks in the ampulla of the spinning gland and to assist their transformation into threads on demand [5] . The sequence composition of the NTD is unusual and its fold is unique with no homologue identified so far [7] . Notably, only 9% of NTD amino-acid side chains are ionizable, which is a small number compared with the average 29% in proteins [17] . This is in particular remarkable, as charged side chains on protein surfaces usually provide water solubility. The side chain charges of the NTD are very likely to have additional roles in spidroin assembly because a protonation event at physiological pH triggers NTD self-association in the spinning duct [7] , [9] , [10] . The mechanistic understanding of this process has two aspects: first, the functionality of the pH-sensitive relay that triggers association and, second, the actual association process itself. NTDs dimerize promoted by a decrease of solution pH from 7 to 6 (refs 7 , 9 , 10 ) ( Fig. 1 ). Thus, a protonation event acts on monomeric NTD where it triggers a change of structural and/or physicochemical properties that facilitates subsequent association. The site(s) of protonation in the NTD and the mechanism of the pH relay are not yet established. To lose or take a proton, the pK a s of involved side chains must lie within the range of the applied pH change, that is, between 7 and 6. The normal pK a of carboxylic acids in proteins is 3–4 but strongly depends on the local environment [17] . Proximity of negatively charged carboxylates leads to unfavourable Coulomb repulsion and can elevate their pK a s to physiological value, thus alleviating repulsive Coulomb forces through protonation [17] . Askarieh et al. [7] suggested from the crystal structure of the dimer and mutagenesis experiments that a direct interaction between the D40 and E84 side chain carboxylates could generate a pH relay. However, a subsequent solution NMR study showed significant structural differences between monomeric and dimeric forms of the NTD [13] ( Fig. 6a ). From the solution structure it is evident that the interaction between D40 and E84, which is present in the dimer, is absent in the monomer. This seems to exclude the D40/E84 interaction as a pH relay. Here we deleted all 12 side chain charges of the NTD individually and probed their influence on kinetics of dimerization. From our analysis, it emerges that D39N and D40N are the only mutants that abolish dimerization ( Fig. 5 ). Both mutants had virtually no fluorescence signal change in rapid-mixing experiments ( Fig. 3a ). Mutation E84Q, on the other hand, had only a minor effect. The observed inability of D40N to form dimers is in agreement with results from Askarieh et al. [7] as well as fluorescence and mass spectrometry studies [7] , [18] . However, the effect of mutating D39 was not examined in these previous studies. Results suggests that D39 and D40 may form a pH relay. The side chains of D39 and D40 are fixed on a helix in close spatial proximity, both in monomeric and dimeric NTD ( Fig. 6a ). D39 and D40 may be close enough to elevate their pK a s to physiological value. A mutual pK a -elevating effect would be abolished on mutation of either one of the two side chains to asparagine and protonation-induced dimerization at pH 6 would be abrogated, as observed in our experiments. However, there is an additional side chain that may have a role. E119Q was the only mutation that significantly stabilizes the dimer. The dissociation rate constant of E119Q is fivefold slower than that of the pseudo wild-type protein and provides a stabilizing free energy of 0.7±0.2 kcal mol −1 ( Fig. 5b ). It is conceivable that an elevated side chain pK a of E119 leads to protonation at pH 6, thereby removing the charge of the carboxylate. In support of this interpretation, computer simulations predicted a destabilizing penetration of water molecules into the dimerization interface mediated by the E119 carboxylate [19] . However, experimental evidence for the protonation of specific side chains in the NTD at pH 6 is still incomplete and may eventually come from high-resolution spectroscopic techniques such as NMR [17] , [20] . 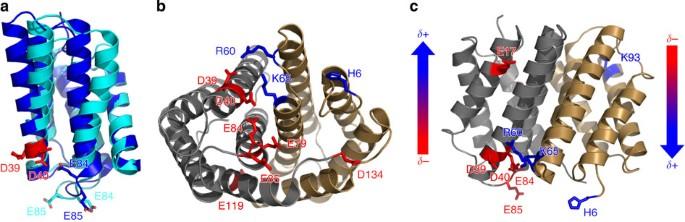Figure 6: Distribution of side chain charges in the NTD. (a) Alignment of the solution structure of monomeric NTD at pH 7 (cyan, pdb id 2LPJ) with the crystal structure of dimeric NTD (blue, pdb id 3LR2) reveals distinct conformational changes13. Shown is a view onto the association interface. Residues D39 and D40 are highlighted in red. Helices of the interface tilt out in the monomer conformation. The structural element surrounding E84 is a coil in the monomer but a helix in the dimer. (b,c) Location of ionizable amino-acid side chains in dimeric NTD (bottom and side view, pdb id 3LR2). The anti-parallel oriented subunits and coloured grey and brown. Acidic (red) and basic (blue) side chains are depicted in stick representation. The macromolecular dipole moment of each subunit that originates from an uneven distribution of side chain charges, identified in structural studies7, is indicated by arrows. Figure 6: Distribution of side chain charges in the NTD. ( a ) Alignment of the solution structure of monomeric NTD at pH 7 (cyan, pdb id 2LPJ) with the crystal structure of dimeric NTD (blue, pdb id 3LR2) reveals distinct conformational changes [13] . Shown is a view onto the association interface. Residues D39 and D40 are highlighted in red. Helices of the interface tilt out in the monomer conformation. The structural element surrounding E84 is a coil in the monomer but a helix in the dimer. ( b , c ) Location of ionizable amino-acid side chains in dimeric NTD (bottom and side view, pdb id 3LR2). The anti-parallel oriented subunits and coloured grey and brown. Acidic (red) and basic (blue) side chains are depicted in stick representation. The macromolecular dipole moment of each subunit that originates from an uneven distribution of side chain charges, identified in structural studies [7] , is indicated by arrows. Full size image Other ionizable side chains also contribute to assembly. We find that mutation of R60 and K65 results in substantial destabilization of the dimer by free energy increments of ~2 kcal mol −1 ( Fig. 5b ). Positively charged R60 and K65 form intersubunit salt bridges with D39 and D40 ( Fig. 6b ). The stabilizing effect of these salt bridges has recently been addressed by computer simulations [21] . We also found that mutation of K93 destabilizes the dimer ( Fig. 5b ). However, this effect is difficult to interpret because the K93 side chain is in a buried position ( Fig. 6c ) and its mutation to alanine may possibly induce a structural perturbation. H6A and E79Q have values of k a and k d that are not substantially different from those of the pseudo wild-type protein. This corroborates findings from previous experimental studies where both mutants were still able to form dimers [7] , [18] . The second question surrounding the mechanism of NTD assembly involves the actual association process itself that follows the protonation event(s). The universal theory of protein–protein association is well established. The shape of most proteins can be approximated as globules and their rates of random collision in aqueous solution is estimated from the Einstein–Smoluchowski equation to ~6 × 10 9 M −1 s −1 at 25 °C (ref. 22 ). Protein association, however, rarely reaches this speed limit set by diffusion. Protein association has strict geometric constraints where complementary shapes require well-defined orientations before they can assemble. The probability of correct orientation of interfaces during a random collision is estimated to ~1.5 × 10 −5 and results in the basal rate constant of protein–protein association of ~10 5 M −1 s −1 (refs 15 , 22 , 23 ). Here we observe an unusually high NTD association rate constant of 3 × 10 8 M −1 s −1 , which is three orders of magnitude faster than the basal value and close to the diffusion speed limit. Favourable intermolecular Coulomb forces originating from opposite charges on protein interfaces can accelerate association to beyond the basal value [15] . This accelerating effect, however, is commonly screened by electrolytes in solution with numerous examples reported in the literature [15] , [16] , [24] , [25] , [26] , [27] , [28] . Surprisingly, we find that association of the NTD is insensitive to such screening ( Fig. 4 ). But IS substantially accelerates NTD dissociation ( Fig. 4 ). This behaviour is the exact opposite of what is commonly observed [15] . Findings are corroborated by results from mutagenesis: deletion of NTD side chain charges have virtually no influence on the rate constant of association but accelerate dissociation ( Fig. 5a,b ). Previous structural studies analysed the distribution of side chain charges on the surface of the NTD [7] . The authors found that opposite charges cluster on opposing poles of the association interface, thereby generating a unique macromolecular dipole [7] . The anti-parallel symmetry of the interface leads to a favourable dipole–dipole interaction ( Fig. 6c ). This dipole interaction may provide the alignment force for accelerated association and explain its unusual insensitivity to dielectric screening. Early simulations on cytochrome c peroxidase emphasized the importance of dipolar interactions as steering force in proteins [29] . Gilson et al. [30] predicted from calculations of protein electrostatics that for many interactions involving dipoles, solvent screening can essentially be ignored. In line with this argument, Lockhart and Kim [31] found experimental evidence that, in contrast to charges, helix dipole interactions in proteins are hardly screened by IS. Findings may have implications in the synthesis of silk fibres by web spiders. For spiders, the speed of dragline synthesis is vital. The fibre is being used both as web frame and the spider’s lifeline. At a vertical fall and during roping, reeling speed can exceed 1 m s −1 (refs 1 , 32 ). At such high reeling speed and rate of fibre synthesis, the residence time of spidroins in the acidified NTD assembly zone of the duct is only about 1 ms depending on spider size. Spidroin NTDs must therefore associate very quickly to assist silk synthesis. The spinning duct of web spiders contains up to 50% spidroin [1] . With a spidroin molecular weight of ~300 kDa, the concentration equals ~1 mM. Together with the basal rate constant of protein–protein association of ~10 5 M −1 s −1 (refs 15 , 22 , 23 ), the concentration yields a basal association time of ~10 ms, which is already too slow for rapid fibre synthesis. The association of the NTD in context of an intact spidroin in the spinning gland may even occur significantly slower than estimated from the basal rate constant of protein association. Although the NTD is an autonomously folded, structurally independent domain it takes only ~5% of a spidroin sequence. Its mobility could additionally be slowed by the presence of the extended repetitive domains that undergo structural transitions in the gland. Moreover, the high spidroin concentration leads to unusual viscid solution properties [1] that will further slow diffusional motions of the NTDs. These considerations emphasize the requirement of accelerated NTD association beyond the basal value if it should assist the process of silk synthesis at high reeling speed. Acceleration by a common charge-driven process would be perturbed by the presence of physiological electrolytes in the spinning duct [34] . In the distal part of the duct where the silk fibre is formed, water is recovered from the spidroin solution [1] , [4] leading to even an increase of IS. A macromolecular NTD dipole interaction that resists dielectric screening could accelerate association irrespective of IS, as observed in our experiments, and thus facilitate the synthesis of dragline silk at high reeling speed. Sequence conservation of NTDs from various silk glands and spider species suggests that such process could be a universal feature of silk fibre synthesis by web spiders. Synthesis and mutagenesis and fluorescence modification of the NTD The complementary DNA of the NTD from spidroin 1 of the major ampullate gland of the nursery web spider E. australis was purchased as synthetic gene, codon optimized for expression in Escherichia coli bacterial cells (GeneArt, Life Technologies). The NTD gene containing an N-terminal His 6 -tag followed by the thrombin recognition sequence (LVPRGS) for proteolytic cleavage was cloned into a modified pRSETA vector (Invitrogen). Single-point mutants were generated using the QuikChange mutagenesis protocol (Stratagene). NTD and mutants thereof were overexpressed in E. coli C41 (DE3) cells and isolated from clarified cell lysate by nickel nitrilotriacetic acid affinity chromatography, followed by proteolytic removal of the His 6 -tag using thrombin from bovine plasma (Sigma). The thrombin-digested eluate from affinity chromatography was dialyzed into 20 mM MES pH 6.0, subsequently applied to an anion-exchange chromatography column (Poros HQ resin equilibrated with 20 mM MES pH 6.0) and eluted with a gradient from 0 to 500 mM sodium chloride. Pooled NTD fractions were purified to homogeneity using size exclusion chromatograpy (SEC) on a Superdex 75 column (GE Healthcare) equilibrated with 200 mM ammonium bicarbonate. The pooled fractions from SEC were lyophilized and stored at −20 °C. NTD-Q50C and mutants thereof were modified with the thiol-reactive maleimide derivative of the oxazine fluorophore AttoOxa11 (Atto-Tec). Labelling was carried out using a 10-fold molar excess of fluorophore reacted for 2.5 h at 25 °C in 50 mM 3-(morpholino)propanesulphonic acid, pH 7.5, containing 6 M guanidinium chloride and a 10-fold molar excess of tris (2-carboxyethyl)phosphine (Sigma) to prevent thiol oxidation. Labelled protein was isolated from unreacted dye using SEC. Steady-state and time-resolved fluorescence experiments Steady-state absorption and fluorescence emission spectra were recorded on a V-650 spectrophotometer and a FP-6500 spectrofluorimeter (Jasco). Association and dissociation kinetics were measured using stopped-flow fluorescence spectroscopy. Trp fluorescence data of NTD were recorded on an Applied Photophysics (SX 18MV) machine equipped with a xenon-lamp as excitation source. AttoOxa11 fluorescence data of NTD F were recorded on a SFM-2000 machine (BioLogic Instruments) using a diode at 639 nm as excitation source. Samples were filtered through 0.2 μm syringe filters before measurement. For determination of k a of NTD, NTD F and mutants thereof, protein samples were prepared at varying concentration in 10 mM MES pH 7.0 with IS adjusted to 150 mM and rapidly mixed into 50 mM MES buffer at pH 6.0 using a volumetric mixing ratio of 1:10. For measurement of k d of NTD F and mutants thereof, 100 nM samples were prepared in 50 mM MES pH 6.0 and chased with 5 μM unlabelled NTD prepared in the same buffer, using a volumetric mixing ratio of 1:10. IS of buffers was adjusted using potassium chloride. All measurements were done at 25 °C. Data analysis Kinetic transients were fitted to exponential decay and rise functions. Values of k a of NTD, NTD F and mutants thereof were determined from the slopes of linear data fits to the concentration dependencies of k obs (five different concentrations each). Values of k d from chasing experiments were determined as average values of observed rate constants from three measurements. The equilibrium dissociation constant, K d , and the free energy of dimerization, Δ G , was calculated from k a and k d : R is the gas constant and T the temperature (298 K). The change of free energy on mutation, ΔΔ G , was calculated by: where K d WT and K d M are the K d values of NTD F (WT) and a single-point mutant (M). How to cite this article: Schwarze, S. et al. The N-terminal domains of spider silk proteins assemble ultrafast and protected from charge screening. Nat. Commun. 4:2815 doi: 10.1038/ncomms3815 (2013).